Tunable quantum beam splitters for coherent manipulation of a solid-state tripartite qubit system Coherent control of quantum states is at the heart of implementing solid-state quantum processors and testing quantum mechanics at the macroscopic level. Despite significant progress made in recent years in controlling single- and bi-partite quantum systems, coherent control of quantum wave function in multipartite systems involving artificial solid-state qubits has been hampered due to the relatively short decoherence time and lack of precise control methods. Here we report the creation and coherent manipulation of quantum states in a tripartite quantum system, which is formed by a superconducting qubit coupled to two microscopic two-level systems (TLSs). The avoided crossings in the system's energy-level spectrum due to the qubit–TLS interaction act as tunable quantum beam splitters of wave functions. Our result shows that the Landau–Zener–Stückelberg interference has great potential in precise control of the quantum states in the tripartite system. As one of three major forms of superconducting qubits [1] , [2] , [3] , a flux-biased superconducting phase qubit [4] , [5] consists of a superconducting loop with inductance L interrupted by a Josephson junction ( Fig. 1a ). The superconducting phase difference ϕ across the junction serves as the quantum variable of coordinate. When biased close to the critical current I 0 , the qubit can be thought of as a tunable artificial atom with discrete energy levels that exist in a potential energy landscape determined by the circuit design parameters and bias ( Fig. 1b ). The ground state |0 and the first excited state |1 are usually chosen as the computational basis states of the phase qubit. The energy difference between |1 and |0 , ω 10 , decreases with flux bias. A TLS is phenomenologically understood to be an atom or a small group of atoms tunnelling between two lattice configurations inside the Josephson tunnel barrier, with different wave functions | L and | R corresponding to different critical currents ( Fig. 1c ). Under the interaction picture of the qubit–TLS system, the state of the TLS can be expressed in terms of the eigenenergy, with | g being the ground state and | e the excited state. When the energy difference between | e and | g , ħω TLS = E e − E g , is close to ℏ ω 10 ( ħ ≡ h /2 π , where h is Planck's constant), coupling between the phase qubit and the TLS becomes significant, which could result in increased decoherence [4] , [5] . On the other hand, one can use strong qubit–TLS coupling to demonstrate coherent macroscopic quantum phenomena and/or quantum information processing [6] , [7] , [8] . For instance, recently, a tetrapartite system formed by two qubits, one cavity and one TLS, has been studied [5] . However, although multipartite spectral property and vacuum Rabi oscillation have been observed, coherent manipulation of the quantum states of the whole system has not yet been demonstrated. 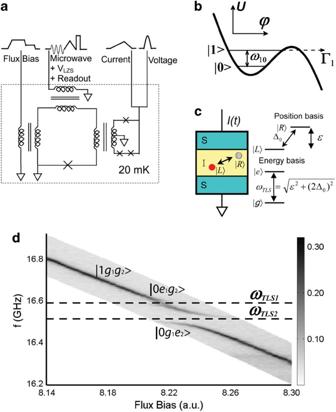Figure 1: Qubit circuit and experimental procedure. (a) Schematic of the qubit circuitry. Josephson junctions Al/AlOx/Al are denoted by the X symbols. The flux bias, microwave and readout dc-SQUID are inductively coupled to the qubit with inductanceL≈770 pH, capacitanceC≈240 fF and critical currentI0≈1.4 μA. (b) Principle of the operation and measurement of the phase qubit. The two lowest eigenstates, |0and |1, form the qubit with transition frequencyω10, which can be adjusted by changing the flux bias. A microwave pulse is used to manipulate the qubit state and readout pulse and then lower the potential energy barrier to perform a fast single-shot readout. (c) Schematic of a two-level state located inside the insulating tunnel barrier of a Josephson junction and its eigenstates in different bases. (d) Spectroscopy of the coupled qubit–TLS system with corresponding quantum states labelled. Two avoided crossings centered atωTLS1andωTLS2are observed. Figure 1: Qubit circuit and experimental procedure. ( a ) Schematic of the qubit circuitry. Josephson junctions Al/AlOx/Al are denoted by the X symbols. The flux bias, microwave and readout dc-SQUID are inductively coupled to the qubit with inductance L ≈770 pH, capacitance C ≈240 fF and critical current I 0 ≈1.4 μA. ( b ) Principle of the operation and measurement of the phase qubit. The two lowest eigenstates, |0 and |1 , form the qubit with transition frequency ω 10 , which can be adjusted by changing the flux bias. A microwave pulse is used to manipulate the qubit state and readout pulse and then lower the potential energy barrier to perform a fast single-shot readout. ( c ) Schematic of a two-level state located inside the insulating tunnel barrier of a Josephson junction and its eigenstates in different bases. ( d ) Spectroscopy of the coupled qubit–TLS system with corresponding quantum states labelled. Two avoided crossings centered at ω TLS1 and ω TLS2 are observed. Full size image In our experiments, we use two TLSs near 16.5 GHz to form a hybrid tripartite [9] , [10] , [11] phase qubit–TLS system and demonstrate Landau–Zener–Stückelberg (LZS) interference in such a tripartite system. The avoided crossings due to the qubit–TLS interaction act as tunable quantum beam splitters of wave functions, with which we could precisely control the quantum states of the system. Experimental results of LZS interference Figure 1d shows the measured spectroscopy of a phase qubit. The spectroscopy data clearly show two avoided crossings resulting from qubit–TLS coupling. As, after application of the π -pulse, the system has absorbed exactly one microwave photon and the subsequent steps of state manipulation are accomplished in the absence of the microwave, conservation of energy guarantees that one and only one of the qubit, TLS1 and TLS2, can be coherently transferred to its excited state. Thus, only as marked in Figure 1d , are involved in the dynamics of the system. Notice that these three basis states form a generalized W state [10] , [11] , [12] , which preserves entanglement between the remaining bipartite system even when one of the qubits is lost and has been recognized as an important resource in quantum information science [13] . The system's effective Hamiltonian can be written as where Δ 1 (Δ 2 ) is the coupling strength between the qubit and TLS1 (TLS2). ω TLS1 ( ω TLS2 ) is the resonant frequency of TLS1 (TLS2). ω 10 ( t )= ω 10,dc − s Φ( t ), with ω 10,dc being the initial energy detuning controlled by the dc flux bias line (that is, the second platform holds in the dc flux bias line), s =|d ω 10 (Φ)/dΦ| being the diabatic energy-level slope of state |1 g 1 g 2 and Φ( t ) being the time-dependent flux bias ( Fig. 1a ). In our experiment, coherent quantum control of multiple qubits is realized with LZ transition. When the system is swept through the avoided crossing, the asymptotic probability of transmission is exp(−2 π (Δ 2 / ν )), where ħν ≡d E /d t denotes the rate of the energy spacing change for noninteracting levels, and 2 ħ Δ is the minimum energy gap. It ranges from 0 to 1, depending on the ratio of Δ and ν . The avoided crossing serves as a beam splitter that splits the initial state into a coherent superposition of two states [14] . These two states evolve independently in time, while a relative phase is accumulated, causing interference after sweeping back and forth through the avoided crossing. Such LZS interference has been observed recently in superconducting qubits [15] , [16] , [17] , [18] , [19] , [20] , [21] , [22] . However, in these experiments the avoided crossings of the single-qubit energy spectrum are used, and microwaves, whose phase is difficult to control, are applied to drive the system through the avoided crossing consecutively to manipulate the qubit state. Here we use a triangular bias waveform with width shorter than the qubit's decoherence time to coherently control the quantum state of the tripartite system. The use of a triangular waveform, with a time resolution of 0.1 ns, ensures precise control of the flux bias sweep at a constant rate and thus the quantum state. The qubit is initially prepared in |0 g 1 g 2 . A resonant microwave π -pulse is applied to coherently transfer the qubit to |1 g 1 g 2 . A triangular flux bias, Φ( t ), with variable width T and amplitude Φ LZS is then applied immediately to the phase qubit to induce LZ transitions ( Fig. 2d ). This is followed by a short readout pulse (about 5 ns) to determine the probability of finding the qubit in the state |1 , that is, the system in the state |1 g 1 g 2 . 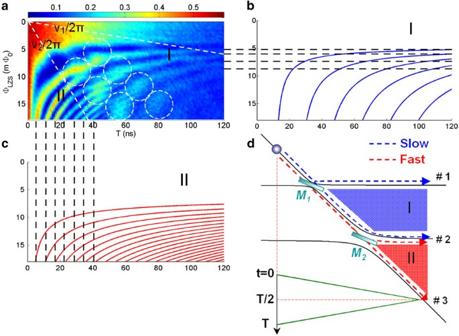Figure 2: LZS interference in a phase qubit coupled to two TLSs. (a) The population of |1measured immediately (a few ns) after the triangular flux pulse is plotted as a function of the width and amplitude of the triangular flux bias waveform. The oblique dotted lines are lines of constant characteristic sweeping rates,ν1andν2, defined in the text. The white circles mark the 'hot spots', where the interference fringes generated byM2tend to fade out and the interference fringes generated byM1dominate. (b,c) Analytically calculated constructive interference strips in regions I and II, respectively. The horizontal and vertical dotted lines indicate the corresponding locations of interference strips. (b,c) have the same axis labels as (a). (d) Schematic of generating LZS interference with tunable beam splitters in a phase qubit coupled to two TLSs.M1andM2correspond to the TLSs with smaller and larger avoided crossings inFigure 1d, respectively. Figure 2: LZS interference in a phase qubit coupled to two TLSs. ( a ) The population of |1 measured immediately (a few ns) after the triangular flux pulse is plotted as a function of the width and amplitude of the triangular flux bias waveform. The oblique dotted lines are lines of constant characteristic sweeping rates, ν 1 and ν 2 , defined in the text. The white circles mark the 'hot spots', where the interference fringes generated by M 2 tend to fade out and the interference fringes generated by M 1 dominate. ( b , c ) Analytically calculated constructive interference strips in regions I and II, respectively. The horizontal and vertical dotted lines indicate the corresponding locations of interference strips. ( b , c ) have the same axis labels as ( a ). ( d ) Schematic of generating LZS interference with tunable beam splitters in a phase qubit coupled to two TLSs. M 1 and M 2 correspond to the TLSs with smaller and larger avoided crossings in Figure 1d , respectively. Full size image Figure 2a shows the measured population of |1 as a function of T and Φ LZS . On the top part of the plot, the amplitude is so small that the state could not reach the first avoided crossing M 1 . Therefore, no LZ transition could occur and only a trivial monotonic behaviour is observed. When the amplitude is large enough to reach M 1 , the emerging interference pattern can be qualitatively divided into three regions with remarkably different fringe patterns. Quantitative comparison with the model To quantitatively model the data, we calculate the probability to return to the initial state P 1 by considering the action of the unitary operations on the initially prepared state. Neglecting relaxation and dephasing, we find where P LZ i ( i =1,2) is the LZ transition probability at the i th avoided crossing M i , and θ I and θ II are the phases accumulated in regions I and II, respectively ( Fig. 2b ). The phase jump at the i th avoided crossing is due to the Stokes phase [16] , [22] θ S i , which depends on the adiabaticity parameter η i =Δ i 2 / ν in the form θ S i = π /4+ η i (ln η i −1)+arg Γ (1− iη i ), where Γ is the Gamma function. In the adiabatic limit θ S →0, while in the sudden limit θ S = π /4. In order to give a clear physical picture, hereafter we adopt the terminology of optics to discuss the phenomenon and its mechanism. First of all we define two characteristic sweeping rates of ν 1 and ν 2 from 2 π Δ i 2 / ν i =1 ( i =1, 2). From the spectroscopy data, we have Δ 1 /2 π =10 MHz and Δ 2 /2 π =32 MHz; thus, ν 1 /2 π =3.94×10 −3 GHz ns −1 and ν 2 /2 π =4.04×10 −2 GHz ns −1 , respectively. These lines of constant sweeping rate characteristic to the system are marked as oblique dotted lines in Figure 2a . The avoided crossings M 1 ( M 2 ) can be viewed as wave function splitters with controllable transmission coefficients set by the sweeping rate ν . ν 1 and ν 2 thereby define three regions in the T −Φ LZS parameter plane that contain all main features of the measured interference patterns: (I) ν ν 1 and ν ν 2 : M 1 acts as a beam splitter and M 2 acts as a total reflection mirror, that is, P LZ1 1/2 and P LZ2 0. In this case, equation (3) can be simplified as Apparently, only path 1 and path 2 contribute to the interference. The phase accumulated in region I can be expressed as where ω i ( t ) ( i =1, 2) denotes the energy frequency corresponding to path i ( i =1, 2). It is easy to find that P 1 is maximized (constructive interference) in the condition from which we can obtain the analytical expression for the positions of constructive interference fringes where δ 1 = ω 10,dc − ω TLS1 , δ 2 = ω 10,dc − ω TLS2 , and δ 12 = ω TLS1 − ω TLS2 . In Figure 2b we show the calculated constructive interference strips, which agree well with the experimental results. Especially, in the limit of s Φ LZS >> δ 2 , δ 12 , equation (7) can be simplified as Intuitively, this result is straightforward to understand, as in the large-amplitude limit the accumulated phase θ 1 is two times the area of a rectangle with length T /2 and width ω TLS1 − ω TLS2 . (II) ν ν 2 and ν >> ν 1 : M 1 acts as a total transmission mirror and M 2 acts as a beam splitter, that is, P LZ1 1 and P LZ2 1/2. In this case, equation (3) can be simplified as Only path 2 and path 3 contribute to the interference. Using the same method in dealing with region I, we obtain the analytical formula governing the positions of constructive interference fringes: As shown in Figure 2c , the positions of the constructive interference fringes obtained from equation (10) agree with experimental results very well. Similarly, in the limit s Φ LZS >> δ 2 , equation (10) has the simple form, which is also readily understood because in the large-amplitude limit the accumulated phase θ II is two times the area of a triangle with base length T /2 and height s Φ LZS . (III) ν 1 < ν < ν 2 : This region is more interesting and complex. Here, M 1 acts as a beam splitter, while M 2 can act either as a beam splitter or as a total reflection mirror. This effect cannot be described by the asymptotic LZ formula because in this region LZS interference occurs only in a relatively small range around the avoided crossings. As the analytical solution is extremely complicated and does not provide clear intuition about the underlying physics, we use a numerically calculated LZ transition probability P LZ corresponding to the transmission coefficient of M 1 and M 2 for comparison with the experimental data. We find that for certain sweeping rates, LZ transition probability resulting from M 2 is quite low. Therefore, M 2 can be treated as a total reflection mirror, while M 1 is still acting as a good beam splitter. The interference fringes generated by M 2 thus disappear (the fringes tend to fade out) and the interference fringes generated by M 1 dominate, displayed as a chain of 'hot spots' marked by the circles in Figure 2a . When both M 1 and M 2 can be treated as beam splitters, all three paths (1, 2, and 3) contribute to the interference. According to equation (3), P 1 is maximized in the condition It is noted that under this condition the term in equation (3) equals 2 nπ . Considering different weights in each path, it is more convenient to obtain a theoretical prediction from a numerical simulation. Here we utilize the Bloch equation to describe the time evolution of the density operator of the tripartite system: where Γ[ ρ ] includes the effects of energy relaxation. 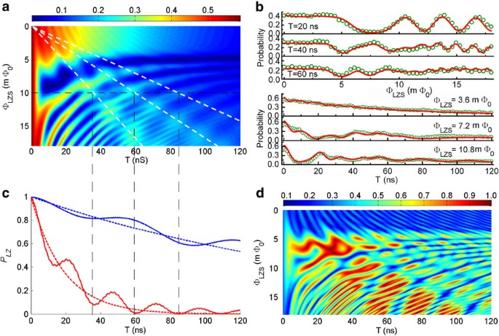Figure 3: Numerically simulated LZS interference pattern and control of a generalizedWstate in a phase qubit coupled to two TLSs. (a) The numerically simulated population of |1after the triangular flux pulse is plotted as a function of the width and amplitude of the triangular flux bias. The horizontal dotted line indicates the location of ΦLZS=10 mΦ0and the vertical dotted lines indicate the locations of 'hot spots' at ΦLZS=10 mΦ0. The oblique dotted lines are lines of constant sweeping rate. The parameters used are determined experimentally:ω01,dc/2π=16.747 GHz,GHz/mΦ0,ωTLS1/2π=16.590 GHz,ωTLS2/2π=16.510 GHz, Δ1/2π=10 MHz, Δ2/2π=32 MHz,γ(deph)=(45ns)−1. (b) The upper panel shows the dependence of population of |1on ΦLZSatT=20, 40 and 60 ns, respectively. The lower panel shows the dependence of population of |1onTat ΦLZS=3.6, 7.2 and 10.8 mΦ0, respectively. The circles represent the experimental data and the lines from the theory. (c) LZ transition probabilities ofM1(blue line) andM2(red line) at ΦLZS=10 mΦ0as a function of pulse width. They are quite different from the asymptotic LZ transition probabilities (blue dotted line and red dotted line). (d) The resultingwas a function ofTand ΦLZS. Figure 3a shows the calculated population of |1 as a function of T and Φ LZS . Figure 3b shows the extracted data for different T and Φ LZS values. The agreement between the theoretical and experimental results is remarkable. In order to better understand the origin of the 'hot spots', we also plot the probabilities of LZ transition as a function of the pulse width at fixed amplitude Φ LZS =10 m Φ 0 ( Fig. 3c ). Notice that both LZ transition probabilities oscillate with T , which are quite different from the general asymptotic LZ transition probabilities. The transition probability at M 1 is always greater because Δ 1 is much smaller than Δ 2 . The three oblique dotted lines in Figure 3a represent lines of constant sweeping rate. The 'hot spots' are located on these lines, where the transition probability of M 2 is a minimum. M 2 thereby acts as a total reflection mirror, resulting in the 'hot spots' in transition probability. This feature further confirms that the avoided crossings play the role of quantum mechanical wave function splitters, analogous to continuously tunable beam splitters in optical experiments. The transmission coefficient of the wave function splitters (the avoided crossings) in our experiment can be varied in situ from zero (total reflection) to unity (total transmission) or any value in between by adjusting the duration and amplitude of the single triangular bias waveform used to sweep through the avoided crossings. Figure 3: Numerically simulated LZS interference pattern and control of a generalized W state in a phase qubit coupled to two TLSs. ( a ) The numerically simulated population of |1 after the triangular flux pulse is plotted as a function of the width and amplitude of the triangular flux bias. The horizontal dotted line indicates the location of Φ LZS =10 mΦ 0 and the vertical dotted lines indicate the locations of 'hot spots' at Φ LZS =10 mΦ 0 . The oblique dotted lines are lines of constant sweeping rate. The parameters used are determined experimentally: ω 01,dc /2 π =16.747 GHz, GHz/mΦ 0 , ω TLS 1 /2 π =16.590 GHz, ω TLS 2 /2 π =16.510 GHz, Δ 1 /2 π =10 MHz, Δ 2 /2 π =32 MHz, γ (deph) =(45 ns ) −1 . ( b ) The upper panel shows the dependence of population of |1 on Φ LZS at T =20, 40 and 60 ns, respectively. The lower panel shows the dependence of population of |1 on T at Φ LZS =3.6, 7.2 and 10.8 mΦ 0 , respectively. The circles represent the experimental data and the lines from the theory. ( c ) LZ transition probabilities of M 1 (blue line) and M 2 (red line) at Φ LZS =10 mΦ 0 as a function of pulse width. They are quite different from the asymptotic LZ transition probabilities (blue dotted line and red dotted line). ( d ) The resulting w as a function of T and Φ LZS . Full size image Precise control of the quantum states in the tripartite system We emphasize that the method of using LZS interference for the precise quantum state manipulation described above is performed within the decoherence time of the tripartite system, which is about 140 ns. Through coherent LZ transition, we can thus achieve a high degree of control over the quantum state of the qubit–TLS tripartite system. For example, one may take advantage of LZS to control the generalized W state, | ψ = α |1 g 1 g 2 + β |0 e 1 g 2 + γ |0 g 1 e 2 , evolving in the sub-space spanned by the three product states during the operation of sweeping flux bias. In order to quantify the generalized W state, we define where σ = α, β, γ . In Figure 3d , w is plotted as a function of T and Φ LZS . Note that with precise control of the flux bias sweep, the states with w =1, which are generalized W states with equal probability in each of the three basis product states, are obtained, demonstrating the effectiveness of this new method. It should be pointed out that when one of the three qubits is lost, the remaining two qubits are maximally entangled. Our tripartite system includes a macroscopic object, which is relatively easy to control and read out, coupled to microscopic degrees of freedom that are less prone to environment-induced decoherence and thus can be used as a hybrid qubit. The excellent agreement between our data and theory over the entire T −Φ LZS parameter plane indicates strongly that the states created are consistent with the generalized W states. The coherent generation and manipulation of generalized W states reported here demonstrate an effective new technique for the precise control of multipartite quantum states in solid-state qubits and/or hybrid qubits [6] , [8] . Experimental detail Figure 1a shows the principal circuitry of the measurement. The flux bias and microwave are fed through the on-chip thin film flux lines coupled inductively to the qubit. The slowly varying flux bias is used to prepare the initial state of the qubit and to read out the qubit state after coherent state manipulation. In the first platform of the flux bias, the potential is tilted quite asymmetrically to ensure that the qubit is initialized in the left well. Then we increase the flux bias to the second platform until there are only a few energy levels, including the computational basis states |0 and |1 in the left well. A microwave π -pulse is applied to rotate the qubit from |0 to |1 . This is followed by a triangular waveform with adjustable width and amplitude applied to the fast flux bias line, which results in LZ transition. A short readout pulse of flux bias is then used to adiabatically reduce the well's depth so that the qubit will tunnel to the right well if it was in |1 or remain in the left well if it was in |0 . The flux bias is then lowered to the third platform, where the double-well potential is symmetric, to freeze the final state in one of the wells. The state in the left or right well corresponds to clockwise or counterclockwise current in the loop, which can be distinguished by the dc-SQUID magnetometer inductively coupled to the qubit. By mapping the states |0 and |1 into the left and right wells, respectively, the probability of finding the qubit in state |1 is obtained. We obtained T 1 70 ns from energy relaxation measurement ( Supplementary Fig. S1a ), T R 80 ns from Rabi oscillation ( Supplementary Fig. S1b ), T 2 * 60 ns from Ramsey interference fringe ( Supplementary Figs S1c and S1d ) and T 2 137 ns from spin-echo ( Supplementary Fig. S1e ) in the region free of qubit–TLS coupling. Hamiltonian in our tripartite system For the coupled qubit–TLS system, the Hamiltonian can be written as [23] , [24] In the two-level approximation the effective Hamiltonian of the qubit is here the flux bias (Φ) dependent energy-level spacing of the qubit, ħω 10 = E 1 − E 0 , can be obtained numerically by solving the eigenvalues problem associated with the full Hamiltonian of the phase qubit [25] . The Hamiltonian of the i th TLS can be written as where ħω TLS i is the energy-level spacing of the i th TLS. The interaction Hamiltonian between the qubit and the i th TLS is where Δ i is the coupling strength between the qubit and the i th TLS and are the Pauli operators acting on the states of the qubit (the i th TLS). By adjusting the flux bias, the qubit and TLSs can be tuned into and out of resonance, effectively turning on and off the couplings. Below |0 and |1 (| g i and | e i ) are used to denote the ground state and excited state of the qubit (the i th TLS). In our experiment the initial state is prepared in the system's ground state |0 g 1 g 2 . When the couplings between the qubit and TLSs are off, we use a π -pulse to pump the qubit to |1 (thus the system is in |1 g 1 g 2 ). We then sweep the flux bias through the avoided crossing(s) to turn on the coupling(s) between the qubit and the TLS(s). Since after the application of the π -pulse the system has absorbed exactly one microwave photon and the subsequent steps of state manipulation are accomplished in the absence of the microwave, conservation of energy guarantees that one and only one of the qubit, TLS1 and TLS2, can be coherently transferred to its excited state. Therefore, states with only one of the three subsystems in excited state, |1 g 1 g 2 , |0 e 1 g 2 , and |1 g 1 e 2 , are relevant in discussing the subsequent coherent dynamics of the system. In the subspace spanned by these three basis states, the Hamiltonian (14) can be written explicitly as Hamiltonian (1) in the main text. Unitary operation in our tripartite system We use the transfer matrix method [16] , [22] to obtain the probability of finding the system in |1 g 1 g 2 at the end of the triangular pulse. We use | a =[1,0,0] T , | b =[0,1,0] T and | c =[0,0,1] T to denote the instantaneous eigenstates of the time-dependent Hamiltonian (14), as shown in Supplementary Figure S2 . It is noted that at the initial flux bias point, which is far from the avoided crossings, the system is in | a =|1 g 1 g 2 . At the crossing times t = t 1 and t = t 2 , the incoming and outgoing states are connected by the transfer matrix: and respectively. Here sin 2 ( θ i /2)= P LZ i ( i =1, 2) is the LZ transition probability at the i th avoided crossing. where θ Si is the Stokes phase [16] , [22] , the value of which depends on the adiabaticity parameter η i =Δ i 2 / υ in the form of θ Si = π /4+ η i (ln η i −1)+arg Γ (1−i η i ), where Γ is the Gamma function. In the adiabatic limit θ S →0, and in the sudden limit θ S = π /4. At crossing times t = t 3 and t = t 4 , we have respectively. The outgoing state at t = t i and the incoming state at t = t i +1 ( i =0, 1, 2, 3, 4) are thus connected by the propagator where ω i ( t ) is the energy-level spacing frequency of | i ( i=a , b , c ) at time t . The net effect of a triangular pulse is to cause the state vector to evolve according to the unitary transformation The probability of finding the system remaining at the initial state is P 1 =| 1 g 1 g 2 | Û |1 g 1 g 2 | 2 . Its concrete form is equation (3), in which and are the relative phases accumulated in regions I and II, respectively, as shown in Supplementary Fig. S2 . The LZS in our experiment can be viewed as interferences among the three paths, which are labelled 1, 2 and 3, starting from the same initial state: path 1: path 2: path 3: Denoting ω i ( t ) as the energy-level spacing frequency corresponding to path i ( i =1, 2, 3), then θ I and θ II have the forms and respectively. Numerical simulation of LZS interference in the bipartite qubit–TLS system For the bipartite qubit–TLS system discussed here, the qubit is coupled only to a single TLS. The quantum dynamics of the system, including the effects of dissipation, is described by the Bloch equation of the time evolution of the density operator: where where ω 10 ( t )= ω 10,dc − νt , ν ≡2 s Φ LZS / T is the energy sweeping rate and Δ is the qubit–TLS coupling strength. The second term, Γ [ ρ ], describes the relaxation process to the ground state |0 g and dephasing process phenomenologically. In a concrete expression, equation (19) can be written as (for ease of discussion, we relabel |1 g and |0 e as | a and | b , respectively) with ρ ba = ρ ab *. Here Γ α ( α = a , b ) is the relaxation rate from state | α to the ground state |0 g . The decoherence rate includes contributions from both relaxation and dephasing. Supplementary Figures S3a and S3b give the numerically simulated LZS interference pattern for the qubit coupled with the first TLS and second TLS, respectively. To calculate the transmission coefficient of M i ( i =1, 2), that is, the LZ tunneling probability P LZ , as shown in Figure 3c , we cannot directly use the asymptotic LZ formula, which is based on sweeping the system across the avoided crossing from negative to positive infinities. In contrast, in our experiment the LZS occurs near the avoided crossings. Therefore, our numerical results are obtained by solving the Bloch equations directly. Numerical simulation of LZS interference in the tripartite qubit–TLS system For the tripartite qubit–TLS system discussed below, the qubit is coupled resonantly to two TLSs (TLS1 and TLS2) with different excited state energies ħω TLS1 and ħω TLS2 . The Hamiltonian in the basis of |1 g 1 g 2 , |0 e 1 g 2 , |0 g 1 e 2 is Hamiltonian (1) in the main text. The Bloch equations that govern the evolution of the density operator can be written as (for simplicity, we relabel respectively) where the diagonal elements ρ ii are the populations, off-diagonal elements ρ ij ( i ≠ j ) describe coherence, and are the rates of decoherence. The remaining three elements' equations are determined by ρ ij *= ρ ji . The numerically simulated LZS interference pattern is shown in Figure 3a , which agrees with the experimental results excellently. How to cite this article: Sun, G. et al . Tunable quantum beam splitters for coherent manipulation of a solid-state tripartite qubit system. Nat. Commun. 1:51 doi: 10.1038/ncomms1050 (2010).